Ultra-high mobility transparent organic thin film transistors grown by an off-centre spin-coating method Organic semiconductors with higher carrier mobility and better transparency have been actively pursued for numerous applications, such as flat-panel display backplane and sensor arrays. The carrier mobility is an important figure of merit and is sensitively influenced by the crystallinity and the molecular arrangement in a crystal lattice. Here we describe the growth of a highly aligned meta-stable structure of 2,7-dioctyl[1]benzothieno[3,2-b][1]benzothiophene (C8-BTBT) from a blended solution of C8-BTBT and polystyrene by using a novel off-centre spin-coating method. Combined with a vertical phase separation of the blend, the highly aligned, meta-stable C8-BTBT films provide a significantly increased thin film transistor hole mobility up to 43 cm 2 Vs −1 (25 cm 2 Vs −1 on average), which is the highest value reported to date for all organic molecules. The resulting transistors show high transparency of >90% over the visible spectrum, indicating their potential for transparent, high-performance organic electronics. Transparent organic semiconductors with high charge-carrier mobilities have been an important research target due to their broad applications in flat-panel displays [1] , [2] , radio-frequency identification tags [3] , [4] , complementary integrated circuits [5] , [6] , [7] and biological and medical applications [8] , [9] , [10] , [11] , [12] , [13] . The carrier mobility of organic semiconductor films is strongly influenced by the crystallinity, molecular packing structures of the organic thin films and charge traps at the gate dielectric/semiconductor interface [14] , [15] , [16] , [17] . Because of the small van der Waals interaction between organic molecules, the crystallinity, grain size and crystal alignment of the solution-processed organic thin films have been shown to be very sensitive to the fabrication conditions, such as solvent evaporation rate [18] , and liquid surface tension force [19] , [20] . In addition to the changed thin film morphology, certain molecular organic semiconductors can form various molecular packing structures (polymorphs) by changing film formation processes [19] , [20] . Since the electronic wavefunction overlap that determines the charge transfer integral is a very sensitive function of the precise molecular packing, the various polymorphs generally have different carrier mobilities with some having a higher mobility than their equilibrium structures [10] , [19] , [20] , [21] , [22] , [23] . In this manuscript, we report the formation of a highly aligned, meta-stable crystal packing structure (likely a polymorph) of 2,7-dioctyl[1]benzothieno[3,2-b][1]benzothiophene (C8-BTBT by a simple off-centre spin-coating (OCSC) method, wherein C8-BTBT and polystyrene (PS) blend solution was used to result in simultaneously a passivation effect of the dielectric surface as well as improving the continuity of the thin C8-BTBT film. An ultra-high maximum hole mobility of 43 cm 2 Vs −1 and an average hole mobility of 25 cm 2 Vs −1 were obtained, much higher than the previously reported average hole mobility of 3~16 cm 2 Vs −1 (refs 18 , 24 , 25 , 26 ). OCSC and device transparency The organic thin film transistors (OTFTs) were fabricated on either highly doped silicon substrates or transparent indium tin oxide (ITO) coated glass substrates with a bottom-gate top-contact structure ( Fig. 1a ). A crosslinked poly(4-vinylphenol) (PVP) was used as the gate dielectric layer ( Supplementary Fig. 1 ) [27] . The semiconductor channel layer was deposited by an OCSC method, in which the substrate is placed away from the centre of the spin-coater ( Fig. 1b and Supplementary Fig. 2 ), using a blend of C8-BTBT with an insulating PS. Since all the organic materials used here have large bandgaps, the resulting films when cast on ITO substrates showed an excellent transparency of >90% in the visible region ( Fig. 1c ), which is comparable to the best transparencies reported to date for TFTs, including both organic and metal oxide TFTs [28] , [29] . Such highly transparent transistors are of great interest for flat-panel display backplane and sensor array applications. 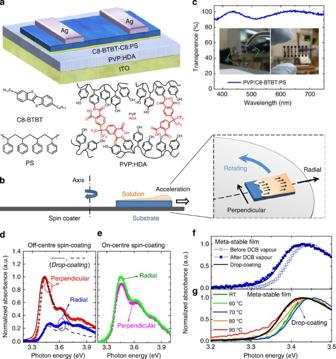Figure 1: Highly aligned meta-stable C8-BTBT:PS film fabricated by OCSC method. (a) Schematic device configuration of OTFT with C8-BTBT:PS blends as channel layer, PVP:HDA as dielectric layer and ITO as the gate electrode; the chemical structures of C8-BTBT, PS, PVP and HDA are shown. (b) Schematic illustration of the OCSC process, in which the substrates are located away from the axis of the spin-coater. (c) Transmission spectrum of the PVP:HDA/C8-BTBT:PS film. Inset: photographs of C8-BTBT:PS film and corresponding OTFT device with a structure of glass/ITO/PVP:HDA/C8-BTBT:PS. (d) Normalized polarized-absorption spectrum of OCSC C8-BTBT:PS film, where the light electrical field is in radial (blue circles) or perpendicular direction (red circles). The two directions are marked in the Fig. 1b; for comparison, the absorption peak of C8-BTBT film prepared by small-angle drop-coating, according to literature procedures25, is also shown (d,f,g, dark line). (e) Normalized polarized-absorption spectrum of on-centre spin-coated C8-BTBT:PS film, where the light electrical field is in radial (green circles) or perpendicular direction (pink circles). (f) Perpendicular polarized-absorption spectrum of meta-stable C8-BTBT:PS film before and after DCB vapour annealing. (g) Perpendicular polarized-absorption spectrum of meta-stable C8-BTBT:PS film after thermal annealing for 3 h at each temperature. Figure 1: Highly aligned meta-stable C8-BTBT:PS film fabricated by OCSC method. ( a ) Schematic device configuration of OTFT with C8-BTBT:PS blends as channel layer, PVP:HDA as dielectric layer and ITO as the gate electrode; the chemical structures of C8-BTBT, PS, PVP and HDA are shown. ( b ) Schematic illustration of the OCSC process, in which the substrates are located away from the axis of the spin-coater. ( c ) Transmission spectrum of the PVP:HDA/C8-BTBT:PS film. Inset: photographs of C8-BTBT:PS film and corresponding OTFT device with a structure of glass/ITO/PVP:HDA/C8-BTBT:PS. ( d ) Normalized polarized-absorption spectrum of OCSC C8-BTBT:PS film, where the light electrical field is in radial (blue circles) or perpendicular direction (red circles). The two directions are marked in the Fig. 1b; for comparison, the absorption peak of C8-BTBT film prepared by small-angle drop-coating, according to literature procedures [25] , is also shown ( d , f , g , dark line). ( e ) Normalized polarized-absorption spectrum of on-centre spin-coated C8-BTBT:PS film, where the light electrical field is in radial (green circles) or perpendicular direction (pink circles). ( f ) Perpendicular polarized-absorption spectrum of meta-stable C8-BTBT:PS film before and after DCB vapour annealing. ( g ) Perpendicular polarized-absorption spectrum of meta-stable C8-BTBT:PS film after thermal annealing for 3 h at each temperature. Full size image Formation of highly aligned meta-stable C8-BTBT films In the OCSC process, the centrifugal force is almost unidirectional over the whole substrate. This method produced highly aligned C8-BTBT crystals, as confirmed by their distinct anisotropic optical absorption spectra under varying polarization of incident light. The peak absorbance of the C8-BTBT film formed by the OCSC method is 2.5 times stronger when the light polarization direction is perpendicular to the radial direction as compared with the radial direction ( Fig. 1d ). In contrast, the C8-BTBT films fabricated by conventional on-centre spin-coating (i.e., substrate centre sitting at the centre of spin-coater axis) showed nearly isotropic light absorption, indicating that crystals in the film were randomly oriented in the plane of the substrate ( Fig. 1e ). There was a small spectral shift of ~50 meV between the peak positions of the first absorption band for the two different polarizations in the OCSC film ( Fig. 1d ), which corresponds to the Davydov splitting of the lowest energy transition in the isolated molecule induced by the anisotropic crystal environment. The C8-BTBT crystals formed by the OCSC method all have a small but distinct blue shift of ~20 meV in the absorption spectrum onset as compared with C8-BTBT crystals prepared through other methods, such as small-angle drop-coating ( Fig. 1d and Supplementary Methods ) [18] , [30] . The spectral differences are indicative of a change in the crystal packing of C8-BTBT. To test whether the OCSC film has a meta-stable crystal structure, we measured absorption spectra before and after solvent vapour annealing ( o -dichlorobenzene, DCB, Fig. 1f ) and thermal annealing (90 °C for 3 h, Fig. 1g ). Both processes resulted in a red-shift of the absorption onset, and the shifted spectra become similar to the spectra obtained from small-angle drop-cast films ( Supplementary Methods ). In addition, we observed that the spectra of the OCSC films were unchanged after being stored at room temperature for more than 1 month ( Supplementary Fig. 3 ) or being annealed at temperatures below 80 °C for 3 h, indicating a long lifetime for the meta-stable film ( Fig. 1g ). Interestingly, it was also noticed that the preferred growth direction of the OCSC film is along the (010) direction of the C8-BTBT crystal ( Supplementary Note 1 and Supplementary Fig. 4 ), which is different from what previously reported, i.e., (100) or (110) directions being the preferred growth direction [24] , [25] . To further support the meta-stable phase and the high crystallinity of C8-BTBT, we performed two-dimensional (2D) grazing incidence X-ray diffraction (GIXD) experiments. The observation of an 18th order out-of-plane (11L) Bragg peak from the OCSC processed thin film (10–20 nm) strongly indicated the highly crystalline nature of our films ( Fig. 2a ) [18] . The in-plane coherence length by Scherrer analysis provided a lower bound crystallite size of ~100 nm. This crystal coherence length is a lower bound value, as sample degradation and peak broadening occurred with X-ray beam exposure ( Supplementary Fig. 5 ). In contrast, the Bragg peaks of the on-centre spin-coated C8-BTBT films were generally broader, with peak widths corresponding to smaller crystallite sizes (<20 nm). Moreover, in the on-centre spin-coated films, GIXD intensities on the right and left sides of the image are identical, confirming that the crystallites form a 2D powder in the plane of the substrate. In contrast, the observed asymmetric pattern in the OCSC film ( Supplementary Fig. 6 and Supplementary Note 2 ) is an indication of the strong in-plane alignment, and is consistent with the optical absorption spectra. Strong evidence for a new crystal packing structure is derived from the presence of an additional diffraction peak near the (002) Bragg reflection, where the lower Q z ~0.44 Å −1 is in agreement with the (002) plane spacing reported for the equilibrium crystal [31] , while the higher Q z ~0.46 Å −1 is strong evidence for a new polymorph ( Fig. 2b ). This higher Q z peak is from a meta-stable phase since it disappears, or decreases in intensity, after thermal annealing ( Fig. 2b and Supplementary Fig. 7 ). In addition, the clear (11L) Bragg peaks shift in position after thermal annealing ( Fig. 2c ) from Q xy =1.34 Å −1 (meta-stable) to 1.32 Å −1 (equilibrium), indicating a smaller intermolecular spacing along (110) direction in the meta-stable phase. The peak shift has previously been observed for other meta-stable systems as well [19] . The meta-stable (002) Bragg ( Q z ~0.46 Å −1 ) peak is also present in the on-centre spin-coated samples; however, the crystallite size is too small to give high hole carrier mobilities. Unfortunately, we are unable to obtain the crystal structure for these meta-stable films due to beam degradation of the sample upon long X-ray exposure times required to get accurate meta-stable peak positions and intensities ( Supplementary Fig. 5 ). 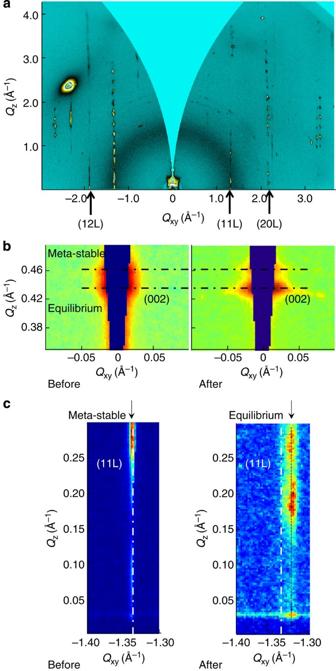Figure 2: GIXD investigations of highly aligned, meta-stable C8-BTBT films. (a) GIXD images of an OCSC C8-BTBT samples. The presence of the asymmetric pattern is indicative of a high degree of in-plane alignment. The high order Bragg peaks indicate good crystallinity. There is an artifact due to the substrate atQxy=−2.1 Å−1andQz=2.1 Å−1. (b) GIXD images of the (002) Bragg peaks of OCSC C8-BTBT:PS film obtained before and after thermal annealing, where the peak related to the meta-stable phase (top peak,Qxy~0.46 Å−1) is less intense compared with that from the equilibrium phase (bottom peak,Qxy~0.44 Å−1) after the thermal anneal. (c) GIXD images of the (11L) Bragg peaks of OCSC C8-BTBT:PS film obtained before and after thermal annealing. The in-plane position of (11L) Bragg peaks shifted after the film was heated to above 90 °C and was subsequently cooled down to room temperature. The (11L) Bragg peaks first disappeared while the (00L) peaks remained visible, indicating the formation of a liquid crystalline phase (Supplementary Fig. 7b). The (11L) Bragg peaks then reformed as the film was cooled, but the (11L) peak shifted away from the original position, implying that the Bragg peak before heating was caused by a meta-stable phase. Figure 2: GIXD investigations of highly aligned, meta-stable C8-BTBT films. ( a ) GIXD images of an OCSC C8-BTBT samples. The presence of the asymmetric pattern is indicative of a high degree of in-plane alignment. The high order Bragg peaks indicate good crystallinity. There is an artifact due to the substrate at Q xy =−2.1 Å −1 and Q z =2.1 Å −1 . ( b ) GIXD images of the (002) Bragg peaks of OCSC C8-BTBT:PS film obtained before and after thermal annealing, where the peak related to the meta-stable phase (top peak, Q xy ~0.46 Å −1 ) is less intense compared with that from the equilibrium phase (bottom peak, Q xy ~0.44 Å −1 ) after the thermal anneal. ( c ) GIXD images of the (11L) Bragg peaks of OCSC C8-BTBT:PS film obtained before and after thermal annealing. The in-plane position of (11L) Bragg peaks shifted after the film was heated to above 90 °C and was subsequently cooled down to room temperature. The (11L) Bragg peaks first disappeared while the (00L) peaks remained visible, indicating the formation of a liquid crystalline phase ( Supplementary Fig. 7b ). The (11L) Bragg peaks then reformed as the film was cooled, but the (11L) peak shifted away from the original position, implying that the Bragg peak before heating was caused by a meta-stable phase. Full size image Since sample degradation currently precludes the full solution of the unit cell and molecular packing, we additionally characterized our highly aligned films using Near-edge X-ray Absorption Fine-Structure (NEXAFS) Spectroscopy. 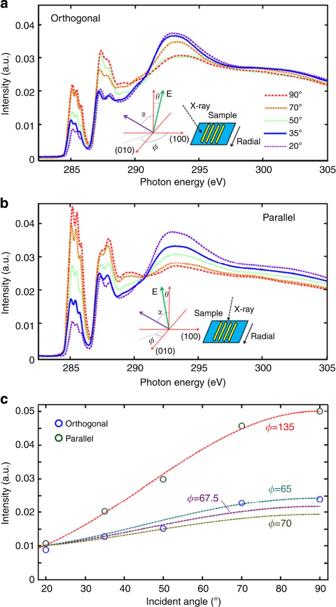Figure 3: NEXAFS investigations of C8-BTBT in-plane alignment. (a) Carbon K edge NEXAFS spectra for the C8-BTBT:PS films at different X-ray incidence angles (θ, i.e., the angle between the X-ray electric fieldEand the normal direction of the substrate plane, where an incident angle of 90° means the incident electric field is in the plane of the substrate. The orientation of the TDM is defined by the polar tilt angleαand the azimuthal angleφ). The lower energy features centred around 285 eV correspond to electronic transitions from core orbitals to antibonding π* orbitals, whereas the higher energy feature centred around 293 eV correspond to the transitions to unbound σ* orbitals. Inset illustration shows the incident electric field of the polarized X-ray is orthogonal to the radial direction. (b) Corresponding NEXAFS spectra for the C8-BTBT:PS films with the incident electric field of the polarized X-ray being parallel to the radial direction. (c) Intensities of the π* transitions versus incidence angle. π* peaks were spectrally integrated from 283.0 to 286.3 eV, which is shown for both relative sample orientations (orthogonal and parallel) with respect to the incident polarization. The dash lines are the fitting curves with different azimuthal angleφ. Figure 3 shows NEXAFS spectra for C8-BTBT films where the incidence angle of the highly polarized synchrotron X-rays was varied relative to the (100) direction (defined as orthogonal, Fig. 3a and Supplementary Fig. 8 ) and the (010) direction (defined as parallel, Fig. 3b ). Similar results were obtained from C8-BTBT:PS films ( Supplementary Fig. 9 ). The peaks near 285 eV correspond to transition from the C1s core-level to antibonding π* orbitals of the conjugated backbone, where the intensity depends on the angle between the electric field vector and the direction of the final state (π*) orbitals [32] . The data show significant incident angular dependence and azimuthal anisotropy (difference between the two different sample orientations with respect to the beam). This shows a large degree of molecular order, an up-right geometry (the π* signal is strongest at 90°), and an overall in-plane crystal alignment (the π* signal is strongest with electric field vector along radial direction). The observed high in-plane alignment in NEXAFS is consistent with the anisotropic optical absorption spectra ( Fig. 1d ) and GIXD images ( Supplementary Fig. 4 ). In Fig. 3c , the integrated π* intensity from 283.0 to 286.3 eV is plotted versus the incidence angle of the parallel and orthogonal condition, respectively. By comparison with simulations according to the formalism for anisotropic NEXAFS intensity for a π* vector outlined by Stohr and Outka [32] , a transition dipole moment (TDM) tilt angle (the angle between TDM and the normal direction of substrate plane, Supplementary Fig. S8 ) of about 88±3° was obtained. ( Supplementary Figs 9,10 and Supplementary Note 3 ). This is larger than that of the on-centre spun samples, which gave a TDM tilt angle of 77~81 o ( Supplementary Fig. 11 ), suggesting a different molecular packing structure between off-centre spun films and conventionally on-centre spun films. Figure 3: NEXAFS investigations of C8-BTBT in-plane alignment. ( a ) Carbon K edge NEXAFS spectra for the C8-BTBT:PS films at different X-ray incidence angles ( θ , i.e., the angle between the X-ray electric field E and the normal direction of the substrate plane, where an incident angle of 90° means the incident electric field is in the plane of the substrate. The orientation of the TDM is defined by the polar tilt angle α and the azimuthal angle φ ). The lower energy features centred around 285 eV correspond to electronic transitions from core orbitals to antibonding π* orbitals, whereas the higher energy feature centred around 293 eV correspond to the transitions to unbound σ* orbitals. Inset illustration shows the incident electric field of the polarized X-ray is orthogonal to the radial direction. ( b ) Corresponding NEXAFS spectra for the C8-BTBT:PS films with the incident electric field of the polarized X-ray being parallel to the radial direction. ( c ) Intensities of the π* transitions versus incidence angle. π* peaks were spectrally integrated from 283.0 to 286.3 eV, which is shown for both relative sample orientations (orthogonal and parallel) with respect to the incident polarization. The dash lines are the fitting curves with different azimuthal angle φ . Full size image Hole mobilities in the OCSC C8-BTBT films We investigated the hole transport characteristics of the OTFTs made with OCSC films ( Fig. 4 ). These films showed an extremely high maximum hole mobility of 43 cm 2 Vs −1 for saturation mobility and 20 cm 2 Vs −1 for linear mobility. The average saturation mobility is 25 cm 2 Vs −1 (in set of Fig. 4f ). It should be noted that strikingly high saturation mobilities of 90~118 cm 2 Vs −1 were observed several times in some samples and the transfer current curves were shown in Supplementary Fig. 13 . However, due to the lack of reproducibility, we report the maximum of 43 cm 2 Vs −1 here as we observed similar value (35~43 cm 2 Vs −1 ) in around 10% of more than 80 devices fabricated. These mobilities are the highest reported values for small-molecular organic semiconductors to date [18] , [19] , [33] , [34] , [35] . The high channel current of these devices has been independently verified by three research laboratories ( Supplementary Fig. 14 ). 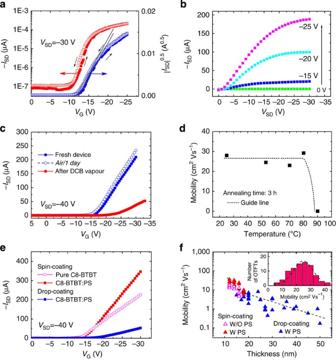Figure 4: High-performance OTFT devices with OCSC C8-BTBT:PS films. (a) Transfer and (b) Output characteristics of an OTFT prepared by OCSC with C8-BTBT:PS film as a channel layer. The channel length is 100 μm, channel width is 1 mm and the capacitance of the dielectric is 1.2 × 10−4F m−2. (c) DCB vapour annealing for 2.5 h decreases the channel current. The channel current for the device kept in air for 1 day is also shown, excluding the possible explanation of device instability. (d) Hole carrier mobilities after thermal annealing for 3 h at each temperature. (e) Comparison of channel current of OTFT with OCSC channel layer or large-angle drop-coated channel layer. (f) Influence of the channel layer thickness and PS blending on the hole mobility. Inset: mobility distribution of the OCSC-prepared OTFTs. Figure 4: High-performance OTFT devices with OCSC C8-BTBT:PS films. ( a ) Transfer and ( b ) Output characteristics of an OTFT prepared by OCSC with C8-BTBT:PS film as a channel layer. The channel length is 100 μm, channel width is 1 mm and the capacitance of the dielectric is 1.2 × 10 −4 F m −2 . ( c ) DCB vapour annealing for 2.5 h decreases the channel current. The channel current for the device kept in air for 1 day is also shown, excluding the possible explanation of device instability. ( d ) Hole carrier mobilities after thermal annealing for 3 h at each temperature. ( e ) Comparison of channel current of OTFT with OCSC channel layer or large-angle drop-coated channel layer. ( f ) Influence of the channel layer thickness and PS blending on the hole mobility. Inset: mobility distribution of the OCSC-prepared OTFTs. Full size image The higher mobilities we obtained here is unlikely to be only attributed to a larger grain size as compared with previous studies, where single crystals were used in the channels [18] , [24] , [25] . Several additional factors may be contributing to the extremely high mobility: the highly aligned crystalline thin film, more continuous formation of C8-BTBT film due to the presence of the PS layer, passivation effect of the PS and possibly the meta-stable packing structure. While our films are highly aligned ( Fig. 3 and Supplementary Figs 4,15 ), the higher mobility values do not originate from the intrinsic anisotropic change transport in the C8-BTBT crystal. This is because the mobilities along the radial and perpendicular directions were measured to be the same in absence of visible grain boundaries or cracks ( Supplementary Fig. 16 ). The observed isotropic mobility is reasonable because the charge transfer integrals along different directions are roughly balanced [16] , [24] . However, the high degree of alignment will still be a contributing factor to the high mobility value because such an alignment reduces the grain boundary scattering [30] . The hole mobility of C8-BTBT has a strong dependence on the film thickness. Two coating methods, OCSC and large-angle drop-coating, were used to tune the C8-BTBT thickness within a range of 10–50 nm. The OCSC films have typical thicknesses from 10 to 18 nm, while the large-angle drop-coating films are around 15–50 nm. In contrast to the formation of the thick C8-BTBT crystals film in Figs 1b , a much larger tilting angle was used in the large-angle drop-coating process to reduce the C8-BTBT thickness to be 15–50 nm ( Supplementary Methods ). Independent of the two coating method, thinner films resulted in higher mobilities ( Fig. 4e,f ) in both cases, while the OCSC films showed the highest mobilities. Second, we observed that blending PS into C8-BTBT yielded significantly higher mobilities ( Fig. 4e,f and Supplementary Fig. 17 ). The higher mobility with PS may be due to enhanced inter-grain connectivity, because the increased solution viscosity helped to form more continuous films, as has been observed with other small molecule/polymer blends [36] , [37] . Another important contributing factor is the vertical phase separation, which generally occurs in polymer and small molecule blends [36] , [38] and would result in reduced surface traps in our devices. To verify the vertical phase separation between C8-BTBT and PS, we studied the films with transmission electron microscopy (TEM) cross-sectional images, where the samples were prepared by being embedded in epoxy resin and microtomed into 70-nm-thick slices. In conventional (unfiltered) cross-sectional TEM view ( Fig. 5a ), the C8-BTBT film is visible as a dark thin layer, due to its high crystallinity and electron density. An additional thinner layer (≤5 nm) is visible in places between the C8-BTBT layer and the substrate, which we attribute to the PS layer. We further confirmed the existence of this ultrathin PS layer by using energy-filtered TEM ( Fig. 5b ). The 22±4 eV image utilized the plasmon peak of the p-type organic semiconductor to enhance the contrast in the electron energy loss spectra, and the thickness map is obtained from the ratio of unfiltered and filtered image, yielding pixel by pixel values of t / λ , where t is film thickness in nanometre and λ is the electron mean free pathway. Both the 22±4 eV image and the thickness map suggest that there is indeed an additional layer underneath C8-BTBT [39] , [40] . Further indication of vertical phase separation in the C8-BTBT:PS film was observed by scanning electron microscopy using a thicker film with a higher percentage of PS, showing a similar phase-separated structure, where the PS layer was sandwiched between the C8-BTBT and PVP film ( Fig. 5c ). The vertical phase separation between C8-BTBT and PS is explained by their different surface energies. The PS segregation to the PVP surface is energetically more favourable than the segregation of C8-BTBT to the PVP surface, because the methyl-terminated C8-BTBT has lower surface energy than either PVP or PS ( Supplementary Note 4 ). 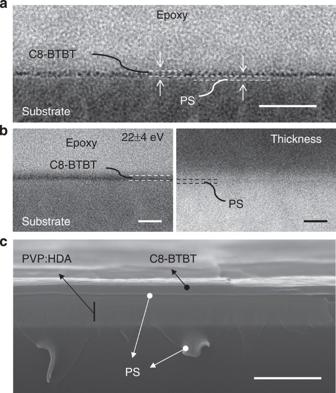Figure 5: Vertical phase separation between C8-BTBT and PS. (a) Cross-sectional TEM of C8-BTBT:PS film without energy filtering. In an unfiltered cross-sectional TEM view, C8-BTBT film is visible as a dark thin layer with 10–20 nm thickness, due to its high crystallinity and electron density. The scale bar is 100 nm. (b) Cross-sectional TEM of C8-BTBT:PS film with energy filtering. Both 22±4 eV image and thickness map suggest that there is an additional layer underneath C8-BTBT. The two scale bars are 50 nm. (c) Cross-sectional scanning electron microscopy (SEM) image of thick C8-BTBT:PS film drop coated on PVP surface, where the PS is more flexible than the C8-BTBT crystal and extended out of the cross section, demonstrating the PS segregation is energetically more favourable than the C8-BTBT segregation to the PVP surface. The scale bar is 1 μm. Figure 5: Vertical phase separation between C8-BTBT and PS. ( a ) Cross-sectional TEM of C8-BTBT:PS film without energy filtering. In an unfiltered cross-sectional TEM view, C8-BTBT film is visible as a dark thin layer with 10–20 nm thickness, due to its high crystallinity and electron density. The scale bar is 100 nm. ( b ) Cross-sectional TEM of C8-BTBT:PS film with energy filtering. Both 22±4 eV image and thickness map suggest that there is an additional layer underneath C8-BTBT. The two scale bars are 50 nm. ( c ) Cross-sectional scanning electron microscopy (SEM) image of thick C8-BTBT:PS film drop coated on PVP surface, where the PS is more flexible than the C8-BTBT crystal and extended out of the cross section, demonstrating the PS segregation is energetically more favourable than the C8-BTBT segregation to the PVP surface. The scale bar is 1 μm. Full size image Covering the PVP surface with an ultrathin layer of PS could reduce the interface traps caused by the polar hydroxyl groups on the PVP chain, contributing to the observed higher mobility [41] , [42] . Previously, the higher mobility in small molecule/polymer blends was also attributed to the ‘zone refinement effect’ during the vertical phase separation process, and this purification effect may also be present in this case [43] , [44] . Furthermore, the lower dielectric constant of PS ( ε r =2.6) than PVP ( ε r =4.2) provides a less polar environment at the dielectric/C8-BTBT interface, leading to a less energetic disorder in the dielectric [45] . Both effects are expected to result in a higher OTFT mobility. Finally, the meta-stable molecular packing in the OCSC film is also a contributing factor to the high mobility as can be seen from the much higher mobility of OCSC film compared with the similarly highly aligned drop-cast film ( Supplementary Table 1 ). The presence of meta-stable packing was clearly supported by the peak shift in GIXD and the relaxation of the peak and shifting of the absorption spectrum to the equilibrium phase features. However, its contribution was difficult to quantify. For example, solvent annealing caused relaxation of the meta-stable polymorph ( Figs 1f,g and 2c ) accompanied by a hole mobility drop from ~26 cm 2 Vs −1 to below 4.1 cm 2 Vs −1 ( Fig. 4c,d ). However, the crystal alignment was also disrupted ( Supplementary Fig. 7 ), making it difficult to attribute the mobility drop entirely to crystal structure change. Moreover, the beam damage during GIXD measurements made it impossible to obtain the precise crystal packing structure for the meta-stable polymorph. Therefore, we were not able to determine the impact of the meta-stable packing on transfer integral. It is not surprising that the ultra-high mobility achieved in the OCSC films combines the contributions from multiple effects. At current stage, it is difficult to pin-point the contribution of each factor quantitatively. Given that we measured very high hole carrier mobilities in TFTs with highly aligned meta-stable C8-BTBT films, it is important to verify that the devices are robust with respect to bias stress. The performance of OTFTs fabricated with meta-stable C8-BTBT film was found to be quite stable under DC bias at room temperature. A source-drain current of 100 μA can be maintained under a DC gate bias of −15 V for over 1,000 s ( Fig. 6 ), which indicates that the meta-stable C8-BTBT films did not undergo a relaxation to the equilibrium phase during continuous current flow. In addition, the low bias stress effect also indicates a negligible trap density in meta-stable C8-BTBT films, which can be attributed to the highly crystalline nature of the film and the presence of few grain boundaries as well as the interfacial trap passivation by the ultrathin PS layer [41] , [42] , [46] , [47] . After a bias stress of over 200 s, the threshold voltage started to decrease ( Fig. 6a , inset). The origin of this shift is not yet fully understood; we hypothesize that this could be related to the motion of ions in the organic layer or the adsorption of moisture at the crosslinked PVP/C8-BTBT interface [48] , [49] . But the I SD difference caused by the continuous bias becomes negligible when the I SD exceeds 10 μA. The transistor also showed good cycle stability under repeated gate voltage pulses (~1 Hz). The I SD remains constant after 750 cycles of switching ( Fig. 6b ). Podzorov and coworkers [50] have shown that the measured hole mobility of C8-BTBT is highly dependent on the gate voltage sweep rate: slowing down the gate voltage sweep rate decreased the mobility from 1 cm 2 Vs −1 to 0.05 cm 2 Vs −1 . This sweep rate-dependent mobility results from the presence of trap states, which cause a strong concomitant stress bias effect. In this study, the device showed a negligible trap state density and thus robust stress bias stability, and no obvious sweep rate-dependent mobility was observed ( Supplementary Fig. 18 ). 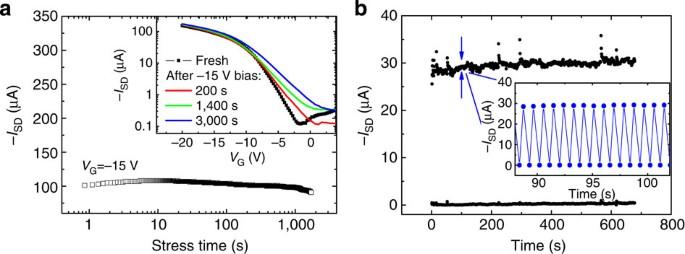Figure 6: Bias stress stability of the high mobility C8-BTBT:PS devices. (a) Stability of the channel current under a continuous bias stress of −15 V for over 1,000 s, inset show theISD-VGcurve taken before and after bias stress. (b) Cycle stability of the device, where a train of gate voltage pulse (−10 V) was applied and the device was switched between on and off for ~750 cycles (1 Hz). Inset show the detailISDresponse at the 90th seconds. Figure 6: Bias stress stability of the high mobility C8-BTBT:PS devices. ( a ) Stability of the channel current under a continuous bias stress of −15 V for over 1,000 s, inset show the I SD - V G curve taken before and after bias stress. ( b ) Cycle stability of the device, where a train of gate voltage pulse (−10 V) was applied and the device was switched between on and off for ~750 cycles (1 Hz). Inset show the detail I SD response at the 90th seconds. Full size image In summary, we have demonstrated a record high hole mobility of 43 cm 2 Vs −1 in OCSC C8-BTBT:PS films (the highest value obtained for small-molecular organic semiconductors) with transparency >90% in the visible range. The OCSC films were considerably thinner than what previously studied and have meta-stable structure. These meta-stable films were observed to maintain its structural integrity up to 80 °C, and the subsequent fabricated devices were stable under both DC and AC bias at room temperature. Our data indicate that the obtained very high hole mobility in C8-BTBT:PS blend films mainly results from the highly aligned crystalline grains with a slightly reduced in-plane intermolecular spacing. The obtained mobility also clearly benefited from PS blending via the formation of vertical phase separation, where the PS segregated to the dielectric/semiconductor interface may have helped to reduce interfacial traps. Collectively, this study demonstrates a new method to enhance the performance of OTFTs. The highest obtained hole mobility is comparable to that of the polycrystalline silicon, indicating a bright future for OTFT applications. Device fabrication For the device fabrication, either ITO-coated glass substrates or highly doped silicon wafers were used. The substrates were first scrubbed with a brush dipped in acetone and ultrasoniced in pure water, acetone and isopropyl alcohol, respectively. Then these substrates were dried in oven at 80 °C. After UV-ozone treatment, the ITO layer was covered by a low temperature cross-linkable PVP dielectric layer according to literature procedures [27] . Here 4,4′-(hexafluoroisopropylidene)diphthalic anhydride (HDA) was used as the cross linker. The PVP-HDA layer was spin-coated from a 100 mg ml −1 solution of PVP:HDA (10:1 by wt) in propylene glycol monomethyl ether acetate. The PVP:HDA films were cured at 100 °C for 60 min to promote the cross-linking reaction, resulting in a dielectric layer thickness of ~330 nm and a measured capacitance of 1.2 × 10 −4 F m −2 ( Supplementary Fig. 1 ). The organic semiconductor films were deposited in an nitrogen inert atmosphere on PVP-HDA-coated ITO substrate from a 5 mg ml −1 C8-BTBT (or C8-BTBT:PS) solution in DCB via a OCSC method ( Supplementary Fig. 2a ), where the substrate (15 × 15 mm 2 ) was placed with its centre away from the rotation axis of the spin-coater at a distance of 20–40 mm. During the OCSC process, the spin speed was gradually increased to 2,700 r.p.m. ( Supplementary Fig. 2b ). The C8-BTBT crystals grow gradually from one side to the other side in the radial direction. The sample was brought out of the N 2 -golve box immediately after spin-coating. The C8-BTBT:PS semiconductor layer fabricated on the PVP surface had an thickness of 10–18 nm, which was varied by changing both spin-coating speed and the solution concentration. Finally, silver (Ag) source and drain electrodes were thermally evaporated through a Si shadow mask with a channel length of 100 μm and a channel width of 1 mm, respectively. The electrical characteristics of the devices were measured with two computer-controlled Keithley 2400 source metre in ambient conditions. Polarized absorption spectroscopy measurement For the polarized absorption spectrum measurements, the C8-BTBT (or C8-BTBT:PS) films were spin coated on PVP:HDA covered quartz with a size of about 25 × 25 mm 2 . Absorption was measured with a UV-Visible spectrophotometer (Thermo Scientific, Evolution 201) combined with a polarizer. The size of the light spot was about 1 × 3 mm 2 . The stability of the meta-stable C8-BTBT:PS film was characterized by optical absorption spectroscopy with the polarization of light in the perpendicular direction ( Supplementary Fig. 3 ). The absorption spectrum of the meta-stable C8-BTBT:PS film was collected multiple times over the course of 1 month storage, during which the C8-BTBT:PS film was kept in the dark at ambient conditions. All the optical measurements were carried out on the same region of the film, with a positional error of about 1~2 mm. GIXD measurement GIXD was performed at the Stanford Synchrotron Radiation Lightsource (SSRL) on beamlines 11-3 and 7-2. The photon energy was 12.73 keV in beamline 11-3 and 8 keV in beamline 7-2. The scattering intensity was recorded on a 2D image plate (MAR-345) with a pixel size of 150 μm (2,300 × 2,300 pixels), located at a distance of either 150 mm or 400 mm from the sample centre for beamline 11-3, and with a point detector for beamline 7-2. The distance between the sample and the detector was calibrated using lanthanum hexaboride (LaB 6 ) polycrystalline standard (beamline 11-3). The incidence angle was chosen in the range of 0.10°–0.14°. The beam size was 50 × 150 μm (vertically and horizontally), which resulted in a 150 μm wide beam footprint on the sample that spanned the length of the 2~3 mm sample. The data were distortion-corrected (theta-dependent image distortion introduced by planar detector surface) before performing quantitative analysis on the images. Numerical integration of the diffraction peak areas was performed with the software WxDiff [51] . The overall resolution in the GIXD experiments, largely determined by the sample size (2-3 mm), was about 0.01 Å −1 . NEXAFS measurement NEXAFS measurements were performed at the bending magnet beamline 8-2 of SSRL [52] , with a ring current of 500 mA, operating the spherical grating monochromator with the 500 l mm −1 grating at intermediate (~0.3 eV) resolution. The toroidal refocusing optics provided a near circular beam cross-section of about 1 mm FWHM (full width at half maximum) in diameter (footprint horizontally was 1–3 mm FWHM pending on the incidence angle). All the samples were mounted in a single load to an aluminium sample holder using conductive carbon, and all the measurements were performed at room temperature and under ultra-high vacuum conditions (below 10 −8 Torr). Both the total electron yield and the Auger electron yield were recorded by means of the sample drain current (measured via a stanford research systems (SRS) current amplifier without bias) and a φ 15–255 G double-pass cylindrical mirror analyser operated in pulse counting mode and at a fixed kinetic energy of 257 eV at 200 eV pass energy. Total electron yield was chosen for the analysis in this work. After dark current subtraction, the sample current was normalized to the incoming photon flux, recorded from a freshly Au-evaporated gold mesh that intercepts ~20% of the beam upstream of the chamber. A linear pre-edge background signal was then subtracted, and the spectra were normalized to the total area. The polarization factor P (defined as the ratio of the in-plane component to the total intensity) of the elliptically polarized synchrotron radiation was assumed to be 90% (ref. 32 ). TEM Measurement For cross-section TEM experiments, the sample films were embedded in low viscosity epoxy and microtomed into thin slices with a thickness of 50–100 nm. TEM experiments were performed in a Zeiss Libra 120 which is equipped with an in-column energy filter. An acceleration voltage of 120 kV was used along with an emission current as small as 5 × 10 −6 A and a minimal beam intensity to avoid electron beam induced morphological change. To examine the nanomorphology of C8-BTBT:PS films across the thickness direction, cross-sectional TEM samples were prepared by embedding the sample films in epoxy resin and microtoming into 70-nm-thick slices. How to cite this article: Yuan, Y. et al . Ultra-high mobility transparent organic thin film transistors grown by an off-centre spin-coating method. Nat. Commun. 5:3005 doi: 10.1038/ncomms4005 (2014).